ATM specifically mediates repair of double-strand breaks with blocked DNA ends Ataxia telangiectasia is caused by mutations in ATM and represents a paradigm for cancer predisposition and neurodegenerative syndromes linked to deficiencies in the DNA-damage response. The role of ATM as a key regulator of signalling following DNA double-strand breaks (DSBs) has been dissected in extraordinary detail, but the impact of this process on DSB repair still remains controversial. Here we develop novel genetic and molecular tools to modify the structure of DSB ends and demonstrate that ATM is indeed required for efficient and accurate DSB repair, preventing cell death and genome instability, but exclusively when the ends are irreversibly blocked. We therefore identify the nature of ATM involvement in DSB repair, presenting blocked DNA ends as a possible pathogenic trigger of ataxia telangiectasia and related disorders. Deficiencies in the DNA-damage response (DDR) are the cause of several human genetic syndromes [1] . Common hallmarks of these disorders include neurodegeneration and/or cancer predisposition, which are a probable consequence of deficient and inaccurate repair of DNA damage. Ataxia telangiectasia (A-T), a rare autosomal recessive syndrome that results from inactivation of the PIKK family Ser/Thr protein kinase ATM (A-T Mutated), is perhaps the paradigm for diseases of this type [2] , [3] . It is characterized by a symptomatology that includes progressive cerebellar ataxia, immunodeficiency, radiosensitivity, hypogonadism and increased cancer incidence (mainly leukaemia and lymphoma). Multiple functions have been assigned to ATM and its list of phosphorylation substrates is extensive [4] . Despite this versatility, its main function, or at least the best understood, is to trigger the initial phosphorylation wave of the DDR to double-strand breaks (DSBs). This fact, together with the exquisite radiosensitivity displayed by ATM-deficient cells and individuals and the symptomatological overlap of A-T with other break repair-defective human syndromes, strongly suggests a link between DSBs and pathology in A-T patients [3] , [5] . On the basis of all of this, one could anticipate that ATM would be essential, or at least important, for the repair of DSBs. Strikingly, this is not the case, as ATM loss does not result in obvious defects in the DSB repair rate. It has therefore been proposed that the radiosensitivity and chromosomal instability observed in ATM-deficient cells more likely arises from deficient checkpoint allowing cell cycle progression in the presence of damaged DNA [6] . However, there is a subset of DSBs, 10–20% depending on the DNA-damaging agent used [7] , [8] , which do require ATM. The current understanding is that these DSBs correspond to damage occurring in heterochromatin, where ATM is required to open the chromatin structure, allowing access of the repair machinery [9] . Interestingly, in addition to this, ATM is involved in specialized DSB-repair mechanisms that are not heterochromatin associated, such as V(D)J, class-switching and meiotic recombination [10] , [11] , [12] . These processes are related to important aspects of A-T pathogenesis such as immunodeficiency, increased incidence of lymphoma and sterility. Fully understanding the nature of DSBs that specifically require ATM for repair could therefore provide important clues into disease pathogenesis. DSBs can harbour different types of chemical moieties that differ from the canonical 5′ phosphate and 3′ hydroxyl at the ends [13] . Cells are therefore endowed with a wide variety of enzymatic activities that can ‘unblock’ DSBs preparing them for repair. However, under certain circumstances, such as the presence of complex or staggered lesions, these activities may be compromised or overwhelmed, resulting in breaks that are ‘blocked,’ in which case the only possibility to allow repair involves the action of nucleases to ‘process’ the ends by cleaving DNA sequence. It is therefore conceivable that clean and blocked DSBs can have different repair requirements and consequences. However, the study of how DNA-end complexity influences the DDR and repair has been traditionally impeded by the heterogeneity in the breaks induced by most DNA-damaging agents. A particular source of DNA breaks is the abortive activity of DNA topoisomerase II (TOP2, α and β isoforms) [14] , which are essential homodimeric enzymes that relax, unknot and/or decatenate DNA molecules [15] . The α isoform is specific to cycling cells, having essential functions during replication and chromosome condensation and segregation. In contrast, the TOP2β is the main TOP2 isoform in quiescent cells and acts mainly in transcription. Despite the important function of TOP2 in essential processes of chromosome metabolism, its mechanism of action can be dangerous, as it involves the passage of duplex DNA through a transient DSB created by the enzyme. This key intermediate of TOP2 activity (termed cleavage complex), in which two topoisomerase subunits are covalently linked to each 5′-terminus of a DSB via a phosphodiester bond between the active-site tyrosine and the 5′-phosphate, is normally very short-lived, because the topoisomerase rapidly religates the DSB once DNA strand passage through the gap has occurred. However, under certain circumstances, such as the presence of nearby DNA lesions, cleavage complexes can be stabilized and interfere with the transcription or replication machinery. If this is the case, trapped TOP2 is degraded, leading to the formation of irreversible DSBs with peptidic blockages at the 5′ ends of the DNA. This mechanism underlies the clinical efficacy of a widely used class of antitumour agents that ‘poison’ topoisomerase activity (for example, etoposide) [16] , thereby prolonging the half-life of the intermediate and increasing the possibility of DSB formation [16] . Etoposide can therefore be used to generate DSBs homogeneously characterized by covalent peptide blockage of the 5′ ends. Tyrosyl DNA phosphodiesterase 2 (TDP2) is the only known enzyme in higher eukaryotes with the physiological capacity to unblock this type of DNA ends, converting them into 5′ phosphate/3′ hydroxyl ligatable termini [17] , [18] , [19] . This scenario offers a unique opportunity for the specific induction of clean and blocked DSBs ( Fig. 1a ). Following etoposide treatment, the majority of the induced DSBs will be efficiently unblocked by TDP2 in wild-type cells. However, when TDP2 is not present, the blockage will be irreversible and will necessarily require alternative nucleolytic processing to allow repair to proceed. This way, clean and blocked DSBs can be specifically induced by etoposide treatment of wild-type and TDP2-deficient cells, respectively. 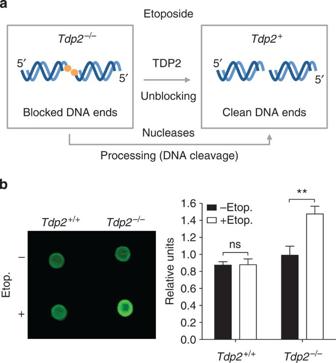Figure 1: Protein-blocked DSBs accumulate inTdp2-deficient background upon TOP2 poison treatment. (a) Scheme of the strategy used to generate breaks with specific structure. (b) SLOPE assay performed inTdp2+/+andTdp2−/−confluency-arrested primary MEFs. Average±s.e.m. of signal from three independent experiments and statistical significance by two-way ANOVA test with Bonferroni post-test is shown (*P≤0.05; **P≤0.01; ***P≤0.001). Figure 1: Protein-blocked DSBs accumulate in Tdp2 -deficient background upon TOP2 poison treatment. ( a ) Scheme of the strategy used to generate breaks with specific structure. ( b ) SLOPE assay performed in Tdp2 +/+ and Tdp2 −/− confluency-arrested primary MEFs. Average±s.e.m. of signal from three independent experiments and statistical significance by two-way ANOVA test with Bonferroni post-test is shown (* P ≤0.05; ** P ≤0.01; *** P ≤0.001). Full size image In this study, we exploit this genetic tool to demonstrate that ATM functions specifically in the rejoining of blocked DSBs, in a manner that is independent of the chromatin status of the lesions. We determine that this novel ATM-dependent repair pathway is particularly relevant for cell survival and the maintenance of genome stability upon induction of blocked DSBs. Finally, we confirm these results using a molecularly defined system and determine that ATM functions in promoting appropriate processing of blocked DSBs. These results put forwards DNA-end structure as a key factor determining ATM involvement during DSB repair, something that could have important implications on our understanding of A-T pathogenesis. Protein-blocked DSBs accumulate in the absence of TDP2 As mentioned above, we can use TOP2 poisons such as etoposide to induce DSBs that are homogeneous in structure. Furthermore, theoretically, we can modulate the ends of these DSBs by working in different genetic backgrounds ( Fig. 1a ): 3′-hydroxyl 5′-phosphate clean ends will be formed in cells containing TDP2 activity, while breaks with a peptide block on 5′ ends will accumulate in TDP2-deficient cells. To validate this experimental setup, we aimed at developing a methodology to specifically measure protein-blocked DSBs, which we have named SLOPE (Selective Labelling Of Protein-blocked Ends). It is based on a previously described assay that has been used to identify genomic regions of TOP2 cleavage [20] . Following isolation of genomic DNA with standard Proteinase K treatment and silica columns, tyrosine residues will remain covalently linked to DNA at the sites of TOP2-blocked DSBs. Biotin is then specifically conjugated to these residues, and finally, the amount of biotin conjugation is measured in dot blots, and used as a specific indicator of protein covalently linked to DNA. To specifically detect irreversible TOP2-blocked DSBs resulting from etoposide treatment, cells are incubated in the absence of the drug to allow cleavage complex reversal before DNA isolation. As can be seen in Fig. 1b , incubation of wild-type primary mouse embryonic fibroblasts (MEFs) with etoposide did not detectably change the amount of protein covalently linked to DNA compared with untreated samples, while a clear and significant increase was observed in Tdp2 −/− cells. These results experimentally demonstrate that, upon etoposide treatment, protein-blocked DSBs accumulate in TDP2-deficient cells, validating our genetic approach for inducing DSBs with different structure. ATM facilitates repair of TOP2-blocked but not clean DSBs We decided to apply the experimental setup described above to analyse the impact of ATM loss on the repair of either clean or blocked DSBs. As an indicator of DSB repair, we followed the time course of Ser139-phosphorylated H2AX (γH2AX) foci disappearance in primary MEFs after etoposide treatment. Since TOP2 activity is subject to cell cycle variations [21] , [22] , cells were confluency arrested to avoid discrepancies in DSB induction. In addition, this simplifies the interpretation of the results, as DSB repair during G0/G1 is limited to non-homologous end-joining [23] . We found that the absence of ATM caused a marked reduction in the intensity of etoposide-induced γH2AX foci ( Supplementary Fig. 1a ); this is not surprising given the key involvement of ATM in H2AX phosphorylation in response to DSBs. However, the number of γH2AX foci per cell was not affected, validating the use of this parameter as a DSB-scoring tool in our setup. In addition, consistent with identical DSB induction, cleavage complexes of TOP2β (the main source of TOP2 activity in quiescent cells [22] ) were also accumulated at similar levels ( Supplementary Fig. 1b ), ruling out an effect of ATM in the generation and processing of TOP2 cleavage complexes. As can be seen in Fig. 2a , the difference in repair rate between Tdp2 +/+ and Tdp2 −/− cells was only minor at the etoposide dose used, which was chosen to avoid artefacts of overwhelming cellular repair capacity. Furthermore, the absence of ATM did not affect the rate of etoposide-induced DSB repair in a TDP2-proficient background. This is consistent with previous observations of a limited DSB-repair defect for IR- but not for etoposide-induced DSBs [8] . ATM, therefore, does not influence repair of clean DSBs. In contrast, a striking drop in the repair kinetics was observed in double Tdp2 −/− Atm −/− cells, with ~40% of the breaks remaining unrepaired even 24 h after induction ( Fig. 2a and Supplementary Fig. 2a ), suggesting that ATM facilitates repair when DSBs are blocked. A single copy of the Tdp2 gene was enough to eliminate blockages, as Tdp2 +/+ and Tdp2 +/− cells were indistinguishable in ATM-deficient background ( Supplementary Fig. 3 ). Importantly, the effect of ATM was specific to TOP2-mediated breaks, not being observed with ionizing radiation ( Supplementary Fig. 2b ), in which case, repair of ~10% of the breaks was ATM dependent, as previously described [7] , but was not affected by TDP2 deficiency. It is worth noting that, as mentioned above, signalling in response to etoposide strongly relies on ATM ( Supplementary Fig. 1a ), but it only has an impact on repair efficiency in the absence of TDP2. Consistent with this independence between signalling and repair, ATM and downstream checkpoint proteins were equally activated in Tdp2 +/+ and Tdp2 −/− cells ( Supplementary Fig. 4 ). 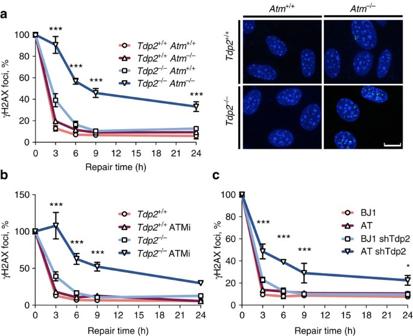Figure 2: ATM facilitates repair of TOP2-blocked DSBs. (a) Time course of γH2AX foci disappearance after 30 min 10 μM etoposide treatment and repair at different times following drug removal inTdp2+/+Atm+/+,Tdp2+/+Atm−/−,Tdp2−/−Atm+/+andTdp2−/−Atm−/−confluency-arrested primary MEFs. Representative images of γH2AX foci (green) and DAPI counterstain (blue) for the 24 h repair time point are shown. Scale bar, 10 μm. (b) As above, inTdp2+/+andTdp2−/−confluency-arrested primary MEFs with or without 10 μM ATM inhibitor (KU55933). (c) As above, in confluency-arrested primary fibroblast derived from A-T patients (AT) and wild-type controls (BJ1) depleted (shTDP2) or not for TDP2. In this case 20 μM etoposide treatment was applied. In all cases, average±s.e.m. of the percentage of foci remaining from at least three independent experiments and the minimal statistical significance between cells deficient in both TDP2 and ATM and all other cells by two-way ANOVA test with Bonferroni post-test is shown (*P≤0.05; **P≤0.01; ***P≤0.001). Figure 2: ATM facilitates repair of TOP2-blocked DSBs. ( a ) Time course of γH2AX foci disappearance after 30 min 10 μM etoposide treatment and repair at different times following drug removal in Tdp2 +/+ Atm +/+ , Tdp2 +/+ Atm −/− , Tdp2 −/− Atm +/+ and Tdp2 −/− Atm −/− confluency-arrested primary MEFs. Representative images of γH2AX foci (green) and DAPI counterstain (blue) for the 24 h repair time point are shown. Scale bar, 10 μm. ( b ) As above, in Tdp2 +/+ and Tdp2 −/− confluency-arrested primary MEFs with or without 10 μM ATM inhibitor (KU55933). ( c ) As above, in confluency-arrested primary fibroblast derived from A-T patients (AT) and wild-type controls (BJ1) depleted (shTDP2) or not for TDP2. In this case 20 μM etoposide treatment was applied. In all cases, average±s.e.m. of the percentage of foci remaining from at least three independent experiments and the minimal statistical significance between cells deficient in both TDP2 and ATM and all other cells by two-way ANOVA test with Bonferroni post-test is shown (* P ≤0.05; ** P ≤0.01; *** P ≤0.001). Full size image To confirm the synergism between Tdp2 and Atm in the repair of etoposide-induced damage during G0/G1, we repeated the analysis but using ATM chemical inhibition instead of deletion ( Fig. 2b and Supplementary Fig. 2c ). As expected, incubation with an ATM inhibitor affected repair of TOP2-induced DSBs in a Tdp2 −/− but not in a Tdp2 +/+ background. This suggests that the role of ATM in the repair of blocked DSBs depends on its kinase activity and rules out artefacts caused by heterogeneity in MEFs. A similar DSB-repair defect was observed when confluency-arrested primary fibroblasts derived from A-T patients were depleted for TDP2 and not in neither wild type nor non-depleted controls ( Fig. 2c and Supplementary Fig. 2d ). In this case, however, the effect was milder, perhaps due to an incomplete knockdown of TDP2, as determined by residual 5′ tyrosyl DNA phosphodiesterase activity ( Supplementary Fig. 2e ). Finally, the effect was not restricted to quiescent cells and was also observed in cycling conditions, both in G1 and G2 stages ( Supplementary Fig. 5 ). Overall, these results constitute strong evidence of an involvement of ATM in DSB repair and suggest that it is specifically linked to DSBs with blocked ends. ATM function on blocked DSBs is heterochromatin independent In the currently accepted model, ATM is specifically required to repair DSBs occurring at heterochromatic regions where it promotes decompaction and facilitates access of the repair machinery [24] . Since TOP2-mediated breakage requires on-going transcription [25] , it should therefore rarely occur within heterochromatin. Thus, we reasoned that the function of ATM in opening chromatin would unlikely account for its involvement in the repair of TOP2-blocked DSBs. In any case, to rule out this possibility, we decided to analyse the location of etoposide-induced γH2AX foci with respect to heterochromatin in Tdp2 −/− Atm −/− confluency-arrested primary MEFs, by three-dimensional confocal microscopy ( Fig. 3 ). As expected, none of the γH2AX foci induced with etoposide colocalized with highly dense chromocenters and only 15.45% (34 out of 220 foci scored) were located at less than 0.4 μm ( Fig. 3a ), which we considered to be heterochromatin associated. In these same conditions, a significantly higher percentage of the breaks (~40%) required ATM activity for their repair ( Fig. 2a ), indicating that the chromatin status of a TOP2-blocked DSB is not a major determinant of ATM requirement for repair. Furthermore, the overall distribution of heterochromatin-associated foci was not significantly changed following 24 h of repair ( Fig. 3b ), with 81.92% of unrepaired foci (154 out of 188) being located within euchromatin ( Fig. 3a ). We conclude that the involvement of ATM in the repair of TOP2-blocked DSBs is largely independent of the reported role of this protein in facilitating repair at heterochromatin regions. 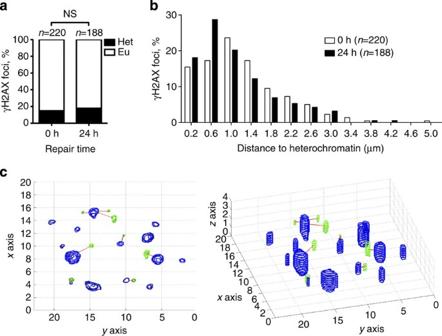Figure 3: Unrepaired TOP2-blocked DSBs are not associated with heterochromatin. Confluency-arrestedAtm−/−Tdp2−/−primary MEFs were treated as described inFig. 1. (a) Percentage of γH2AX foci that are located within heterochromatin (Het) or euchromatin (Eu) following 0 and 24 h repair after etoposide treatment. A cutoff distance of 0.4 μM from the centroid of each focus to the nearest euchromatin/heterochromatin boundary was applied. Statistical significance by Chi Square test is indicated. (b) Distribution of distances between γH2AX foci and heterochromatin as determined above. Bins of 0.4 μm centred on the indicated distance were used for representation. (c) Example of the automatic calculation of distances between γH2AX foci (green) and densely DAPI-stained chromocenters (blue) used for the data shown above. Both a z-stack projection (left) and a 3D reconstitution (right) are shown. Figure 3: Unrepaired TOP2-blocked DSBs are not associated with heterochromatin. Confluency-arrested Atm −/− Tdp2 −/− primary MEFs were treated as described in Fig. 1 . ( a ) Percentage of γH2AX foci that are located within heterochromatin (Het) or euchromatin (Eu) following 0 and 24 h repair after etoposide treatment. A cutoff distance of 0.4 μM from the centroid of each focus to the nearest euchromatin/heterochromatin boundary was applied. Statistical significance by Chi Square test is indicated. ( b ) Distribution of distances between γH2AX foci and heterochromatin as determined above. Bins of 0.4 μm centred on the indicated distance were used for representation. ( c ) Example of the automatic calculation of distances between γH2AX foci (green) and densely DAPI-stained chromocenters (blue) used for the data shown above. Both a z-stack projection (left) and a 3D reconstitution (right) are shown. Full size image ATM function on blocked DSBs has consequences for the cell The incapacity to properly repair a small number or even a single DSB can lead to cell death and/or genome rearrangements. It is therefore conceivable that the DSB-repair defect caused by ATM loss, although affecting a minor fraction of the lesions, underlies the profound radiosensitivity and chromosomal instability observed in A-T patients and cells. We exploited Tdp2 −/− Atm −/− cells to directly address the cellular implications of ATM-linked DSB-repair deficiencies, first by monitoring cell survival in response to etoposide treatment ( Fig. 4a ). Atm deletion in transformed MEFs had a negligible effect on etoposide sensitivity in a wild-type ( Tdp2 +/+ ) background. In contrast, sensitivity of Tdp2 −/− cells, which was mild at this low etoposide doses, was significantly increased by ATM loss, correlating with the observed DSB-repair defect ( Fig. 2a ). An even larger effect was observed if ATM inhibition was used instead of deletion ( Fig. 4b ), confirming the requirement of ATM kinase activity and ruling out differences being caused by heterogeneity intrinsic to the MEFs or the cellular transformation process. Furthermore, the difference observed between deletion and chemical inhibition suggests a possible negative effect of inactive ATM and is consistent with recently observed enhanced phenotypes of catalytically dead ATM [26] , [27] . 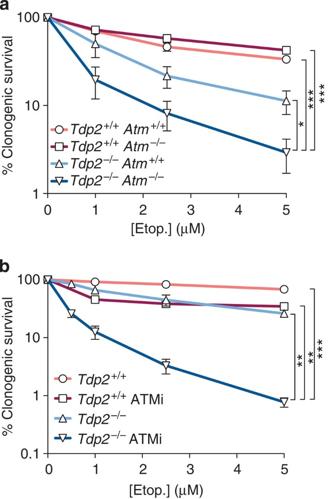Figure 4: ATM promotes survival upon induction of blocked DSBs. (a) Clonogenic survival of the indicated transformed MEFs following acute treatment with the indicated concentrations of etoposide. Average±s.e.m. of at least three independent experiments and statistical significance at the highest indicated dose by one-way ANOVA with Bonferroni post-test are shown (*P≤0.05; **P≤0.01; ***P≤0.001). (b) As above, with or without incubation with 10 μM ATM inhibitor (KU55933). Figure 4: ATM promotes survival upon induction of blocked DSBs. ( a ) Clonogenic survival of the indicated transformed MEFs following acute treatment with the indicated concentrations of etoposide. Average±s.e.m. of at least three independent experiments and statistical significance at the highest indicated dose by one-way ANOVA with Bonferroni post-test are shown (* P ≤0.05; ** P ≤0.01; *** P ≤0.001). ( b ) As above, with or without incubation with 10 μM ATM inhibitor (KU55933). Full size image Furthermore, we addressed the impact of ATM loss on genome integrity following etoposide treatment in Tdp2 +/+ and Tdp2 −/− transformed MEFs. First, we monitored micronuclei formation, which arise from the mis-segregation of chromosomes or acentric chromosomal fragments, and is a well-established indicator of genome instability. To restrict our analysis to micronuclei arising during the cell cycle in which treatment was applied, cytokinesis was blocked with cytochalasin B and only binucleated cells were scored ( Fig. 5a ). Independent deletion of either Atm or Tdp2 caused an increase in etoposide-induced micronuclei. Interestingly, however, the levels were further increased when both genes were simultaneously deleted, doubling the frequency observed in either single mutant. It is worth noting that the frequency observed corresponds to extremely high levels of instability, with many of the cells displaying multiple micronuclei, a qualitative difference compared with single mutants. To confirm these results, we scored chromosomal aberrations in metaphase spreads ( Fig. 5b ). Following etoposide treatment, Tdp2 −/− Atm −/− cells displayed a marked increase in the number of chromosomal aberrations observed. On average, these cells showed a striking 15% aberrant chromosomes, which represent a 7.5-fold and 3-fold increase when compared with single Tdp2 −/− and Atm −/− mutants, respectively. A wide variety of aberration types was observed, including breaks, radial chromosomes and fusions. Overall, these results demonstrate that ATM-mediated repair promotes cell survival and the maintenance of genome integrity in response to blocked DSBs, presenting this particular structure as a possible molecular trigger of important A-T symptoms. One must bear in mind, however, that the cell death and genome instability phenotypes may not be uniquely caused by the blocked DSB-repair defect, but by its combination with a defective checkpoint that allows cell cycle progression in the presence of DNA lesions. 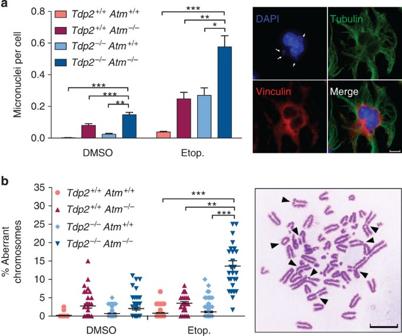Figure 5: ATM promotes the maintenance of genome integrity upon induction of blocked DSBs. (a) Micronuclei were scored in the indicated binucleated transformed MEFs following acute treatment with 2.5 μM etoposide. Histogram bars (left) represent the average±s.e.m. ofn≥600 cells from three independent experiments. Statistical significance by one-way ANOVA with Bonferroni post-test is indicated (*P≤0.05; **P≤0.01; ***P≤0.001). Representative image (right) of a treatedTpd2−/−Atm−/−cell containing multiple micronuclei is shown. Scale bar, 7.5 μm. (b) Chromosomal aberrations (both break and exchange type) were scored following acute treatment with 2.5 μM etoposide. Plot (left) shows the number of aberrations per 100 chromosomes from individual metaphase spreads obtained in at least 6 independent experiments. Average±s.e.m. and statistical significance by Kruskal-Wallis test with Dunn’s post-test is indicated (*P≤0.05; **P≤0.01; ***P≤0.001). Representative image (right) of aTpd2−/−Atm−/−metaphase containing multiple chromosomal aberrations is shown. Scale bar, 10 μm. Figure 5: ATM promotes the maintenance of genome integrity upon induction of blocked DSBs. ( a ) Micronuclei were scored in the indicated binucleated transformed MEFs following acute treatment with 2.5 μM etoposide. Histogram bars (left) represent the average±s.e.m. of n ≥600 cells from three independent experiments. Statistical significance by one-way ANOVA with Bonferroni post-test is indicated (* P ≤0.05; ** P ≤0.01; *** P ≤0.001). Representative image (right) of a treated Tpd2 −/− Atm −/− cell containing multiple micronuclei is shown. Scale bar, 7.5 μm. ( b ) Chromosomal aberrations (both break and exchange type) were scored following acute treatment with 2.5 μM etoposide. Plot (left) shows the number of aberrations per 100 chromosomes from individual metaphase spreads obtained in at least 6 independent experiments. Average±s.e.m. and statistical significance by Kruskal-Wallis test with Dunn’s post-test is indicated (* P ≤0.05; ** P ≤0.01; *** P ≤0.001). Representative image (right) of a Tpd2 −/− Atm −/− metaphase containing multiple chromosomal aberrations is shown. Scale bar, 10 μm. Full size image ATM function on blocked DSBs prevents loss of DNA sequence TOP2-blocked DSBs are only one type of many possible blockages occurring in vivo . We therefore aimed at confirming the involvement of ATM in the repair of blocked DSBs using a different, TOP2-independent, system in which the structure of DNA ends could be molecularly controlled. We started by searching for a 5′ modification that could block DNA ends in vitro . We found that a commercially available 5′-biotin modification was not removed from duplex oligonucleotides in vitro by HEK293T cellular extracts, while clear a 5′ tyrosyl DNA phosphodiesterase activity was observed under the same conditions ( Supplementary Fig. 6a ,b). We decided to use this modification to block the ends of the pEGFP-Pem1 system, which uses reconstitution of GFP expression to measure recircularization of a linear plasmid following transfection into mammalian cells [28] ( Fig. 4a ). Using PCR-mediated amplification with primers with different 5′ end structure, we were able to generate DNA substrates that harboured either clean 5′-phosphates or blocked 5′-biotins at their ends, something that was confirmed by streptavidin-mediated pull-down ( Supplementary Fig. 3c ). As can be seen in Fig. 6b , repair of pEGFP-Pem1 plasmids containing clean 5′-phosphate ends was not significantly affected by incubation of HEK293T cells with an ATM inhibitor, as measured by either the percentage of GFP-expressing cells or the total accumulated GFP fluorescence. In contrast, repair of 5′-biotin containing plasmids was significantly decreased by ATM inhibition, regardless of the quantification method used. As an additional control, we found that ATM was not required to repair a modification such as 5′ hydroxyl that should not result in end blockage due to the existence of cellular machinery to solve the problem (PNKP) ( Supplementary Fig. 6d ). Therefore, by using a molecularly defined system, we confirm that ATM specifically facilitates repair of DSBs that are blocked. 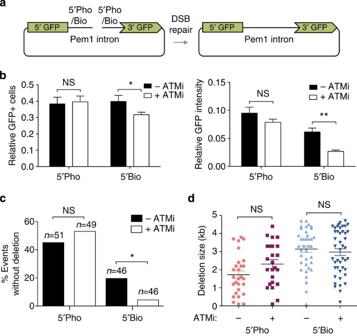Figure 6: ATM facilitates repair of biotin-blocked DSBs. (a) Scheme of the modified pEGFP-Pem1 system harbouring 5′-phosphate or 5′-biotin ends (left) and the expected repair product (right). (b) HEK293T cells were transfected in the presence or absence of 10 μM ATM inhibitor (KU55933) with the substrates described above, and analysed by FACS for GFP-positive cells (left) and average GFP intensity (right). In both cases, data are relative to transfection with a control pEGFP-Pem1 circular plasmid. Average±s.e.m. of four independent experiments and statistical significance by two-way ANOVA with Bonferroni post-test are shown (*P≤0.05; **P≤0.01; ***P≤0.001). (c) Percentage of plasmid-repair events not associated with detectable sequence loss. Statistical significance by Chi Square test is shown (*P≤0.05; **P≤0.01; ***P≤0.001). (d) Deletion size in plasmid repair events. Substrates as described above. Average±s.e.m. and statistical significance by Kruskal-Wallis test with Dunn’s post-test is indicated. Figure 6: ATM facilitates repair of biotin-blocked DSBs. ( a ) Scheme of the modified pEGFP-Pem1 system harbouring 5′-phosphate or 5′-biotin ends (left) and the expected repair product (right). ( b ) HEK293T cells were transfected in the presence or absence of 10 μM ATM inhibitor (KU55933) with the substrates described above, and analysed by FACS for GFP-positive cells (left) and average GFP intensity (right). In both cases, data are relative to transfection with a control pEGFP-Pem1 circular plasmid. Average±s.e.m. of four independent experiments and statistical significance by two-way ANOVA with Bonferroni post-test are shown (* P ≤0.05; ** P ≤0.01; *** P ≤0.001). ( c ) Percentage of plasmid-repair events not associated with detectable sequence loss. Statistical significance by Chi Square test is shown (* P ≤0.05; ** P ≤0.01; *** P ≤0.001). ( d ) Deletion size in plasmid repair events. Substrates as described above. Average±s.e.m. and statistical significance by Kruskal-Wallis test with Dunn’s post-test is indicated. Full size image The system also allows partial loss of sequence at the repair junction thanks to the Pem1 intron (see Fig. 6a ). Thus, not only the quantity, but also the quality of repair can be monitored, something that can provide insights into the mechanisms involved. For this purpose, a minimum of 46 individual events for each condition were cloned in bacteria and subjected to restriction analysis to determine the accuracy of the repair process ( Supplementary Fig. 7 ). Interestingly, ATM inhibitors caused a qualitative change in repair of the 5′-biotin but not the 5′-phosphate substrates, with a marked decrease (from 20% to 5%) in the percentage of repair events not harbouring detectable loss of sequence ( Fig. 6c ). However, in the clones showing DNA loss, the average size of this deleted sequence was unchanged by ATM inhibition ( Fig. 6d ). This demonstrates that ATM prevents excessive sequence loss from DNA ends, which is indicative of its involvement in blocked DSB end processing. Our study demonstrates that ATM is specifically required for the repair of blocked DSBs. With these results in mind, it is tempting to speculate that the observed existence of two subpopulations of DSBs, according to their ATM dependency or independency for repair [8] , to some extent might be based on the structural heterogeneity in the ends induced by DNA-damaging agents. Thus, ATM would not impact in the repair of DSBs with 3′-hydroxyl 5′-phosphate ligatable ends, or those that can be converted into these structures by direct unblocking, while it would greatly facilitate rejoining of DSBs with ends that are blocked and require processing. In addition, we observe that the role of ATM in blocked DSB repair is independent of the chromatin status of the broken DNA, in apparent contradiction with previous observations of a specific role of ATM in the repair of DSBs occurring in heterochromatin [24] . We understand, however, that blocked end and heterochromatin models for ATM involvement in DSB repair are not conflicting, and it is therefore possible to unify both observations if one thinks that ATM is specifically required in conditions in which repair is suboptimal, regardless of the particular molecular reason. Alternatively, it is also possible that heterochromatin, due to its densely packed structure, is more prone to suffer blocked damage, such as clustered DNA lesions and/or DNA-protein crosslinks, than more open regions. It is worth noting that progressive cerebellar ataxia, which is perhaps the most enigmatic (and also debilitating) symptom of A-T, could hardly be explained based on a heterochromatin hypothesis, since the clearest target population in the cerebellum, Purkinje cells, possess a mostly euchromatic nucleus [29] . Our findings change this picture, as blocked DSBs could also occur in Purkinje cells, and could therefore potentially contribute to this aspect of pathology. We would like to clarify that TOP2-mediated DSBs, although successfully used as a tool in this study, may constitute only one particular type of many possible physiological blockages requiring ATM in vivo , and which could, altogether, contribute to A-T pathogenesis. In this sense, ATM has already been directly implicated in two examples of blocked DSB repair with consequences for A-T symptomatology. First, during V(D)J recombination induced by the RAG endonucleases, ATM promotes the stability of coding ends, which are hairpin-blocked, but not of signal ends, which are clean [30] . This deficit likely contributes to immunodeficiency and the development of lymphoid malignancies in A-T [31] . Second, meiotic recombination, which involves the repair of DSBs covalently blocked by the SPO11 protein, is severely compromised in the absence of ATM and is likely the cause of sterility in A-T [10] , [11] . Our results put forward end blockage as a possible molecular explanation for the particular sensitivity of these systems to ATM loss. Finally, it is worth noting that the extreme etoposide sensitivity of double Tdp2 −/− Atm −/− cells opens the door for the use of TDP2 inhibitors, which are currently under development, in sporadic ATM-deficient cancers [32] , [33] , [34] . We envision mainly two complementary manners in which ATM can regulate processing of blocked DSBs ( Fig. 7 ). First, it can promote nucleolytic activity to eliminate the blockage through the action of nucleases such as the MRN complex, CtIP and/or Artemis [8] , [35] , [36] , some of which have already been reported to affect cellular response to etoposide [37] , [38] . Second, it can restrict excessive nucleolytic degradation of DNA ends [39] . This can actually operate by a direct inhibitory action on these same nucleases [40] or others such as EXO1 [41] , and/or by promoting modifications at the DSB, such as for example γH2AX, which can protect from nucleolytic action [42] . This dual impact of ATM on DSB ends, exerted through its wide range of phosphorylation targets, makes it an ideal candidate to orchestrate blocked DSB processing, so it is restricted to the minimal resection necessary to allow rejoining. 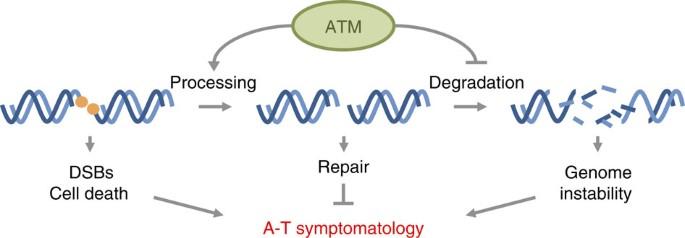Figure 7: Model for ATM involvement in blocked DSB repair. ATM promotes processing of blocked DSBs and inhibits excessive degradation. This promotes efficient and accurate repair, preventing the accumulation of unrepaired DSBs, cell death and genome instability, which can trigger the development of A-T symptomatology. Figure 7: Model for ATM involvement in blocked DSB repair. ATM promotes processing of blocked DSBs and inhibits excessive degradation. This promotes efficient and accurate repair, preventing the accumulation of unrepaired DSBs, cell death and genome instability, which can trigger the development of A-T symptomatology. Full size image In summary, we demonstrate that ATM does indeed function in DSB repair, but specifically to limit the potentially detrimental consequences of blocked DNA ends. If not properly dealt with, these lesions can impact cell survival and genome integrity, which can contribute to the development of A-T symptomatology. Determining the identity of physiologically occurring blockages and their specific influence on pathogenesis should therefore attract future efforts to unravel the aetiology of this devastating disease. Cells and cell culture Primary MEFs were isolated from crosses between Tdp2 −/− and Atm −/− mice [19] , [43] at day 13 p.c. and cultured at 37 °C, 5% CO 2 , 3% O 2 in Dubelcco’s Modified Eagle’s Medium (DMEM) supplemented with penicillin, streptomycin, 15% FCS and non-essential amino acids. All experiments were carried out between P1 and P5. MEFs were transformed by retroviral delivery of T121, a fragment of the SV40 large T antigen that antagonizes the three Rb family members but not p53 (ref. 19 ). Transformed MEFs and HEK293T cells were maintained at 37 °C, 5% CO 2 in DMEM supplemented with penicillin, streptomycin and 10% FCS. A-T (Coriell's Repository GM05823D) and BJ1 primary fibroblasts were cultured at 37 °C, 5% CO 2 , in DMEM supplemented with penicillin, streptomycin and 15% FCS. Selective labelling of protein-blocked DNA ends The selective labelling of protein-blocked DNA ends (SLOPE) assay is a modification of selective labelling of TOP2 cleavage sites (SLOT) protocol [20] . Cells were treated 30 min with 100 μM etoposide or vehicle (DMSO), and 30′ after drug removal (to allow reversal of cleavage complexes) genomic DNA was extracted with the Qiagen Blood and Tissue Kit, which includes proteinase K treatment. Tyrosine residues that remain covalently linked to DNA were labelled with biotin using EDC and amine-PEG3-biotin (Thermo Scientific). DNA was precipitated to eliminate unreacted amine-PEG3-biotin and resuspended in TE buffer. Five hundred nanograms of DNA were dotted on a Hybond-H + (Amersham Bioscience) membrane and cross-linked with 70,000 μJ cm −2 UV. The membrane was blocked with Odyssey blocking buffer (LI-COR Biosciences) with 1% SDS, incubated with IRDye Streptavidin 800CW, 1/10,000 (LI-COR Biosciences) in the same buffer, washed (three times in TBS-0.1% Tween20) and allowed to dry. Dots were analysed and quantified in Odyssey CLx with ImageStudio Odyssey CLx Software. The results are related to an internal control of the same labelling protocol performed on plasmid DNA. Immunofluorescence Cells were grown on coverslips for 7 days until confluency-arrested, treated as indicated and fixed 10 min in ice-cold methanol or 4% PFA-PBS. Cells were then permeabilized (2 min in PBS-0.2% Triton X-100), blocked (30 min in PBS-5% BSA) and incubated with the required primary antibodies (1–3 h in PBS-1% BSA). Cells were then washed (three times in PBS-0.1% Tween 20), incubated for 30 min with the corresponding AlexaFluor-conjugated secondary antibodies (1/1,000 dilution in 1% BSA-PBS) and washed again as described above. Finally, they were counterstained with DAPI (Sigma) and mounted in Vectashield (Vector Labs). γH2AX foci were manually counted (double-blind) in 40 cells from each experimental condition. Primary antibodies were used at the indicated dilution: γH2AX (Millipore, 05-636), 1/1,000; α-Tubulin (Abcam, ab18251), 1/2,000; Vinculin hVIN-1 (Sigma, V9131) 1/2,000. TOPIIβ cleavage complexes Confluency arrested primary MEFs were treated 1 h with 100 μM etoposide or vehicle (DMSO), immediately lysed in 1% Sarkosyl (Sigma) and processed according to the in vivo complex of enzyme (ICE) assay [44] . Samples were centrifuged at 57,000 r.p.m. for 20 h at 25 °C using 3.3 ml 13 × 33 mm polyallomer Optiseal tubes (Beckman Coulter) in a TLN100 rotor (Beckman Coulter). 2.5 μg of precipitated DNA was transferred onto Hybond ECL membranes (GE Healthcare) using a Bio-Dot SF Microfiltration Apparatus (Biorad). Membranes were blocked 1 h with Odyssey Blocking Buffer (LI-COR Biosciences), incubated with 1/1,000 anti-TOP2β antibody (Santa Cruz, sc-13059), in Odyssey Blocking Buffer-0.1% Tween20, washed (three times with TBS-0.1% Tween20), incubated with 1/15,000 IRDye 800CW Goat anti-Rabbit IgG (LI-COR) and finally washed (three times with TBS-0.1%-Tween20 and three times with TBS). Once the membranes were dry, slots were analysed and quantified in Odyssey CLx using ImageStudio Odyssey CLx Software. TDP2 knockdown Lentiviral vectors for TDP2 knockdown (pLKO.1-puro-Tdp2-2; SIGMA, clone TRCN0000003072) and empty control (pLKO.1-puro) were generated in HEK293T transfected with the packaging vectors pCMVDR8.91 and pMDG. A-T and BJ1 primary fibroblasts were infected with pLKO.1-puro-Tdp2-2 or pLKO.1-puro lentiviruses in 100 mm dishes, incubated for 3 days and then placed under puromycin selection (1 μg ml −1 ) for 7 days. 5′ activity in vitro For the preparation of labelled double-stranded 5′-phosphotyrosyl, 5′-phosphobiotin and 5′-phosphate substrates, 5′- TAT ACT TCT CTT TCC AGG GCT ATG T-3′ oligonucleotides with tyrosine (Midland Certified Reagents), biotin (Sigma) or phosphate (Sigma) modifications at the 5′ end were annealed to 5′-AGA CAT AGC CCT GGA AAG AGA AGT ATA-3′ (Sigma) and labelled in the presence of [α-32P]-dCTP, ddTTP and Klenow polymerase. Cell extracts were prepared by mild sonication in Lysis Buffer (40 mM Tris–HCl, pH 7.5, 100 mM NaCl, 0.1% Tween-20, 1 mM DTT) supplemented with 1 mM PMSF and protease inhibitor cocktail (Sigma) followed by clarification 10 min 16,500 g 4 °C. Protein concentration was measured with Bradford reagent (Sigma). 5′ reactions contained 50 nM substrate, 80 μM competitor single-stranded oligonucleotide and the indicated amount of cellular extract in a total volume of 6 μl Reaction Buffer (50 mM Tris–Cl, pH 7.5, 50 mM KCl, 1 mM MgCl 2 , 1 mM DTT, 100 μg ml −1 BSA). Reactions were stopped by the addition of 3 μl 3 × Formamide Loading Buffer and 5 min 95 °C incubation. Samples were resolved by denaturing polyacrylamide gel electrophoresis and analysed by phosphorimaging in a Fujifilm FLA5100 device (GE Healthcare). γH2AX foci in specific cell cycle stages Immunofluorescence was performed as described above with the following modifications. Fixation was performed 10 min at room temperature in 4% PFA-PBS. Cyclin A staining was used to distinguish G1 and S/G2 cells. To exclude replicating cells, 5-ethynyl-2′-deoxyuridine (EdU, Invitrogen) was added throughout treatment and repair at a final concentration of 10 μM. Click chemistry reaction was performed by incubating (30 min r.t.) with 1 μM AlexaFluor 647-conjugated azide (Invitrogen) in reaction cocktail (100 mM TrisHCl pH 8.5, 1 mM CuSO 4 , 100 mM ascorbic acid). γH2AX foci were manually counted (double-blind) in 40 G1 cells (Cyclin A negative) or 20 G2 cells (Cyclin A positive EdU negative) from each experimental condition. Antibodies were used at the indicated dilution: γH2AX (Millipore, 05-636), 1/1,000; Cyclin A (Santa Cruz, sc-751), 1/200. Western blot Confluency-arrested primary MEFs were resuspended on ice using a cell scraper 30 min after treatment with the indicated concentration of etoposide. They were lysed in Laemli buffer and boiled at 96 °C for 5 min. Protein concentration was measured by Pierce 660 nm Protein Assay with Ionic detergent compatibility reagent (Thermo Scientific). Thirty micrograms of sample was run in NuPAGE Tris-Acetate Mini gels 3–8% (Novex) and transferred to Immobilon-FL Transfer Membranes (Millipore). Membranes were blocked in Odyssey Blocking Buffer (LI-COR Biosciences) incubated with primary antibodies in Odyssey Blocking Buffer-0.1% Tween20 and washed (three times in TBS-0.1% Tween20). They were then incubated with the corresponding IRDye-conjugated secondary antibodies in Odyssey Blocking Buffer-0.02% to 0.1% Tween20 and washed (three times in TBS-0.1% Tween20 and 1 × in TBS buffer). Membranes were analyzed in Odyssey CLx with ImageStudio Odyssey CLx Software. Primary antibodies were used at the indicated dilution: ATM (Sigma, MAT3-4G10/8), 1/1,000; ATM pS1981 (Cell Signaling, #4526), 1/1,000; p-CHK2 Thr68 (Cell Signaling, #2661), 1/1,000; p-p53 Ser15 (Cell Signaling, #9284), 1/1,000; p-CHK1 Ser345 (Cell Signaling, #2341), 1/1,000; α-tubulin (Sigma, T9026), 1/50,000. Image processing An in-house MATLAB R2012a-based application was designed to segment nuclei images. For each nucleus, a series of Z-sections (0.21 μm step) were obtained using a Leica TCS-SP5 confocal microscope with a HCX PL APO 63x/1.40λBL objective. These series were segmented to obtain the number, position, intensity and volume values of γH2AX foci and heterochromatin (G and B components of the RGB image, respectively). The segmentation from the different sections was integrated to reconstitute the 3D information of each entire nucleus. Using this reconstitution, the distance between each focus and the nearest euchromatin/heterochromatin boundary in the 3D space was determined. Clonogenic survival assays Survival assays were carried out seeding 2,000 cells in 100 mm dishes, in duplicate for each experimental condition. After 12 h, cells were preincubated with 10 μM ATM inhibitor KU55933 (Tocris) or vehicle for 1 h. The indicated concentration of etoposide was added and cells were incubated for additional 3 h. Following one wash with PBS, fresh medium was added and cells were incubated for 10–14 days. Dishes were fixed and stained for colony scoring in Crystal Violet solution (0.5% Crystal violet in 20% ethanol). The surviving fraction at each dose was calculated by dividing the average number of visible colonies in treated versus untreated dishes. Cytogenetic analysis Micronuclei were analysed in transformed MEFs previously seeded onto coverslips. Following treatment, cytochalasin B (Sigma) was added at 4 μg ml −1 . Twenty-two hours post treatment, cells were fixed and subjected to DAPI staining as described above. Only binucleated cells were scored, which was confirmed by visualization of the cytoplasm with Tubulin and Vinculin immunofluorescence (performed as described above). Chromosomal aberrations were scored in Giemsa-stained metaphase spreads. Following treatment, recovery in fresh medium was allowed for 2 h, and demecolcine (Sigma) was added at a final concentration of 0.2 μg ml −1 . Four hours later, cells were collected by trypsinization, subjected to hypotonic shock for 1 h at 37 °C in 0.3 M sodium citrate, and fixed in 3:1 methanol:acetic acid solution. Cells were dropped onto acetic acid-humidified slides and stained 20 min in Giemsa-modified (Sigma) solution (5% v/v in H 2 O). Validation of pEGF-Pem1 substrates The structure of 5′ DNA ends was analysed by streptavidin-mediated precipitation. Dynabeads (10 μg) M-270 Streptavidin magnetic beads (Invitrogen) were prewashed (3 × in 5 mM Tris–HCl pH 7.5, 0.5 mM EDTA in the presence of 1 M NaCl) and incubated with 100 ng of purified PCR products in the same buffer for 1 h. Beads were then washed 4 × in the same buffer, gradually decreasing NaCl concentration to 0. Finally, DNA was eluted by 2 h incubation with Bgl II restriction enzyme (New England Biolabs) in the recommended buffer. Input, unbound and bound DNA was analysed by agarose gel electrophoresis. Plasmid-circularization assays Substrates were generated by PCR-mediated amplification of plasmid pEGFP-Pem1-Ad2 [28] with primers 5′-AAT TCT TCT CTT TCC AGG GCT AT GT-3′ and 5′- AAT TCA TCC CCA GAA ATG TAA CTT G-3′ harbouring phosphate or biotin moieties at 5′ ends (Sigma). DNA of the correct size was then gel-purified and transfected into HEK293T cells, pretreated for 30 min with 10 μM ATM inhibitor KU55933 (Tocris) or vehicle. Sixteen hours later, cells were analysed by FACS. Individual repair events were cloned in E. coli by plasmid rescue from transfected cells and analysed by digestion with Dra I. Statistical analysis In all cases the indicated statistical test was applied using Prism 5 package (Graphpad). How to cite this article: Álvarez-Quilón, A. et al. ATM specifically mediates repair of double-strand breaks with blocked DNA ends. Nat. Commun. 5:3347 doi: 10.1038/ncomms4347 (2014).